Reputation can enhance or suppress cooperation through positive feedback One possible explanation for the widespread existence of cooperation in nature is that individuals cooperate to establish reputations and so benefit in future interactions with others. We consider a class of games in which individuals contribute to a common good at a cost to themselves. Population members vary in type, that is, in the cost paid for a given level of contribution. We consider a form of indirect reciprocity in which the contribution of an individual depends on their partner’s reputation and their own type. Here we show that for such games, reputation destabilizes the selfish equilibrium through a novel and robust feedback mechanism. For those games in which the selfish optimal contribution to the common good increases as the contribution of the partner increases, the feedback mechanism enhances cooperation levels. In contrast, when the optimal contribution decreases as partner’s contribution increases, cooperation levels are reduced still further. Typically, the members of a natural population vary in their abilities and their behavioural strategies. In particular, there is variation in the degree of cooperativeness when two individuals interact with each other. This raises the possibility that each individual has a different reputation for cooperativeness based on the individual’s behaviour with previous partners. If individuals have reputations that are known to others, it will be advantageous for each population member to take their current partner’s reputation into account in deciding how cooperative to be with that partner. Once population members evolve to so respond, there will then be selection on individuals to change their reputations so as to affect the behaviour of future partners. In this paper, we investigate the effect of this feedback mechanism on the levels of cooperation that evolve in the population. We consider a class of two-player games in which each individual decides how much effort to expend on some common good. The more effort that an individual expends the greater the benefit that each member of the pair derives from the common good, but the greater the cost paid by the focal individual. We divide these games into two classes. In an ‘increasing best-effort’ game, the effort maximizing the payoff to an individual increases as the effort of the partner increases. In a ‘decreasing best-effort’ game, the effort maximizing the payoff on a round decreases as the effort of the partner increases. Games in each class abound in nature. As an example of an increasing best-effort game, consider two fish inspecting a suspicious object that may turn out to be a predator [1] . Here the ‘effort’ of a fish might correspond to the distance the fish advances towards the object. Since it is dangerous to advance alone, the optimal distance to advance increases with the distance advanced by the partner. In situations in which a pair of animals feed together, but must remain vigilant for predators, best efforts will usually be decreasing; the optimal vigilance level of one individual will decrease with the vigilance level of the other [2] . Depending on the biological assumptions, games in which two animals pair up to hunt down prey could potentially be of either type, as could games between parents over care of their young. For such games, we demonstrate a robust mechanism by which cooperation is predicted to evolve. The three key aspects of this mechanism are: A effort levels can vary continuously, B the best behaviour of one individual depends on the behaviour of the opponent, C individuals differ in their payoffs; specifically the marginal cost of a given increase of effort varies between individuals. Although we are concerned with a form of indirect reciprocity [3] , [4] , [5] , [6] , the mechanism is novel because of the role played by individual differences and how this interacts with the other factors. To illustrate this interaction, consider the increasing best-effort case. Note that (c) implies that different individuals will take different actions and hence will differ in their reputation for providing effort. Thus, by (b), it is worth taking note of the partner’s reputation in choosing one’s own effort, and this effort should increase with the partner’s reputation to obtain a higher payoff in the current round. This means that the populations will evolve so that individuals will put in more effort when their partner has a high reputation. This then selects for individuals to increase their effort further so as to enhance their own reputation and hence elicit higher levels of effort from their future partners. This increased effort then leads to selection to increase the effort still further so as to get a high payoff in the current round and so on. In this way, there is a positive feedback leading to high levels of effort. Thus allowing population members to form reputations based on their effort increases levels of cooperation. By analogous reasoning, allowing population members to form reputations in the decreasing best-effort case leads to a feedback process, which reduces the levels of cooperation. To formulate the above verbal arguments mathematically, we consider two game theoretical models (Methods). In one, individuals cannot form reputations. In the other, reputation based on previous effort is possible. In both cases, we find the evolutionarily stable strategy (ESS) in the population and compare the evolutionarily stable (ES) mean population efforts in the two cases, seeing which scenario produces more contribution to the common good. We also compare the above two efforts with the mean effort of a population in which individuals behave so as to maximize the mean fitness of population members (the cooperative solution). In our analysis, the reputation of an individual is an estimate of the mean effort of this individual. A subsidiary aim of the paper is to investigate how the quality of data available to estimate this mean affects the evolved mean population level of effort. As we demonstrate, reputation enhances cooperation for games with increasing best effort and suppresses cooperation for games with decreasing best effort. Furthermore, the effects become more pronounced as the quality of data on the previous behaviour of partner increases. Analytic results To find the ES response rule analytically, we assume that the number of rounds played by an individual is large (we consider the limit as the number tends to infinity). We also Taylor series expand the benefit function, ignoring terms of order 3 and above, and assume that the cost function has a specific quadratic form (Methods). The payoff to an individual is then a quadratic function of the individual’s own effort ( x ) and that of their partner ( y ). In this approximation, the interaction term J is the coefficient of the xy term (Methods). As for the general case (Methods), best responses are increasing when J >0 and are decreasing when J <0. We also assume that the effort of an individual is determined by three genetically determined parameters, m , δ and λ as where v is the individual’s type and r is the opponent’s reputation. Here m is the individual’s baseline effort, δ specifies how responsive the individual is to deviations of their type from the population mean μ and λ specifies their responsiveness to the deviation of the opponent’s reputation from the focal individual’s own baseline effort. For the specified benefits and costs, within the class of rules of the form (1), there is a unique ES rule when there is no reputation (so that λ is constrained to be 0; Supplementary Methods ) and a unique ES rule when reputation is allowed ( Supplementary Methods ). We denote the ES values of m and δ when there is no reputation ( λ =0) by and . Since the mean type of individuals is μ , by equation (1), the ES mean population effort is . We denote ES values of the parameters when individuals are allowed to respond to their opponent’s reputation by m *, δ * and λ *. Since the mean reputation of individuals equals their mean effort (equation (10)), by equation (1), m * is the mean population effort at this evolutionary equilibrium. In Supplementary Methods , we show that the ES values of these various parameters satisfy a number of inequalities. We show that and δ *>0. Thus, in both cases, at evolutionary stability, reputation is an honest signal (with noise) of quality. In the increasing best-effort case, we show that individuals respond positively to the reputation of partner ( λ *>0) and cooperation is enhanced by reputation, that is, where m c is the mean level of effort in a cooperative population. Conversely, when best efforts are decreasing, we show that λ *<0 and cooperation is reduced by reputation, that is, The effect of J and the memory parameter β (Methods) on ES rules are illustrated in Fig. 1 and explored analytically in Supplementary Methods . As the parameter β increases, more weight is put on the more distant past (equation (10)) and estimates of the mean effort of a partner become more accurate. This results in individuals being more responsive to reputation (| λ *| is increased), which accentuates the difference in effort levels between the case of no reputation and that with reputation. 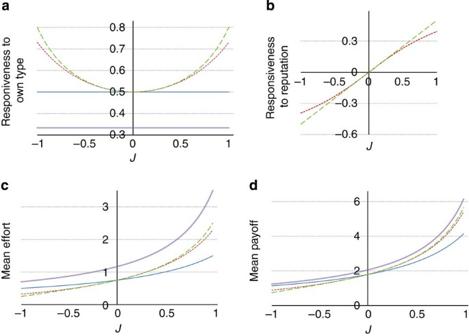Figure 1: Effect of the interaction parameterJon the ES outcome. The benefit function is given byB(x,y)=2(x+y)−0.5(x2+y2)+Jxyand the cost function isCv(x)=vx+0.5x2. (a) Responsiveness to own type (δ). (b) Responsiveness to reputation of partner (λ). (c) Mean population effort. (d) Mean payoff per round. Ina,c,d, the cases considered are (i) there is no reputation (solid line); (ii) reputation is the effort invested on the preceding round (that is,β=0) (dotted line); (iii) reputation is the average effort invested over all previous rounds (that is, the limit asβ→1) (dashed line); (iv) behaviour is cooperative (compound line). Inb, results for cases (ii) and (iii) are shown. Figure 1: Effect of the interaction parameter J on the ES outcome. The benefit function is given by B ( x , y )=2( x + y )−0.5( x 2 + y 2 )+ Jxy and the cost function is C v ( x )= vx +0.5 x 2 . ( a ) Responsiveness to own type ( δ ). ( b ) Responsiveness to reputation of partner ( λ ). ( c ) Mean population effort. ( d ) Mean payoff per round. In a , c , d , the cases considered are (i) there is no reputation (solid line); (ii) reputation is the effort invested on the preceding round (that is, β =0) (dotted line); (iii) reputation is the average effort invested over all previous rounds (that is, the limit as β →1) (dashed line); (iv) behaviour is cooperative (compound line). In b , results for cases (ii) and (iii) are shown. Full size image Evolutionary simulations We supplement the above analytic conclusions with evolutionary simulations in which the parameters m , δ and λ coevolve (Methods). In each evolutionary simulation, for each population member, the parameter λ was held fixed at the value λ =0 for the first 10,000 generations, so that individuals were not allowed to use the reputation of partner. Then after 10,000 generations, λ was allowed to mutate from its value of 0. The analytic analysis is based on the average payoff over infinitely many rounds. To investigate the effect of finitely many rounds, we performed evolutionary simulations in which each population member in each generation played 20 rounds (Methods). 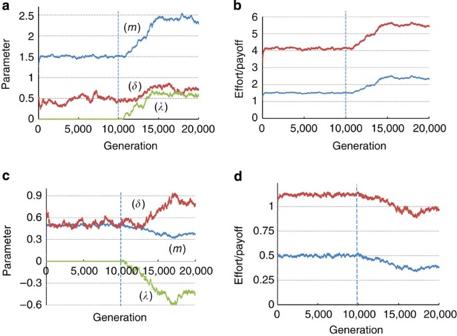Figure 2: Evolutionary simulation results when the benefit and cost functions are as inFig. 1. The parameterλ(responsiveness to reputation of partner) is constrained to be zero until generation 10,000, after which it is allowed to evolve. Ina,b,J=1 so that best efforts are increasing. Inc,d,J=−1 so that best efforts are decreasing.a,cshow population mean values ofm,δandλ(see equation (1)),b,dshow population mean values of the average payoff over all 20 rounds (top curve) and effort on the 20th round (bottom curve).β=0.8 throughout. Figure 2 explores predictions when costs and benefits are the same as in the analytic model. As can be seen, general conclusions still hold when the number of rounds is restricted. Figure 2: Evolutionary simulation results when the benefit and cost functions are as in Fig. 1 . The parameter λ (responsiveness to reputation of partner) is constrained to be zero until generation 10,000, after which it is allowed to evolve. In a , b , J =1 so that best efforts are increasing. In c , d , J =−1 so that best efforts are decreasing. a , c show population mean values of m , δ and λ (see equation (1)), b , d show population mean values of the average payoff over all 20 rounds (top curve) and effort on the 20th round (bottom curve). β =0.8 throughout. Full size image If payoffs are not of the general form assumed in the analytic model, we would not expect unconstrained best-response rules to be linear. Nevertheless, it seems reasonable to assume that evolved simple rules might be approximately linear. Motivated by these considerations, we have evolved linear rules for a variety of benefit and cost functions. 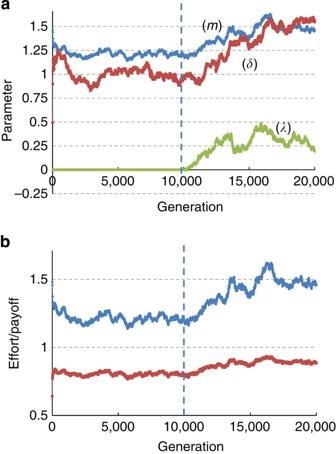Figure 3: Evolutionary simulation results for an increasing best-response case not covered by the analytic model. Benefits and costs areB(x,y)=4xy/[(1+x)(1+y)] andCv(x)=0.1(1+4v)x1.5. (a) Population mean values ofm,δandλ(see equation (1)), (b) population mean values of the average payoff over all 20 rounds (bottom curve) and effort on the 20th round (top curve).β=0.8. Figure 3 shows an example in which the best effort is increasing. Individuals evolve to increase their effort with the reputation of partner, resulting in enhanced mean effort and fitness. 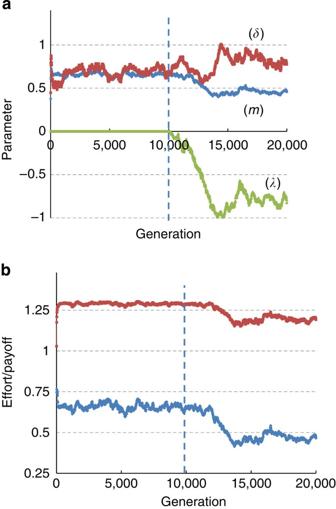Figure 4: Evolutionary simulation results for a decreasing best-response case not covered by the analytic model. Benefits and cost areB(x,y)=2(x+y)/[0.5+x+y] andCv(x)=0.1(1+4v)x1.5. (a) Population mean values ofm,δandλ(see equation (1)), (b) population mean values of the average payoff over all 20 rounds (top curve) and effort on the 20th round (bottom curve).β=0.8. Figure 4 shows an example in which the best effort is decreasing. In this case, efforts evolve to decrease with the reputation of partner, and mean effort and mean fitness is reduced by allowing reputation. Figure 3: Evolutionary simulation results for an increasing best-response case not covered by the analytic model. Benefits and costs are B ( x , y )=4 xy /[(1+ x )(1+ y )] and C v ( x )=0.1(1+4 v ) x 1.5 . ( a ) Population mean values of m , δ and λ (see equation (1)), ( b ) population mean values of the average payoff over all 20 rounds (bottom curve) and effort on the 20th round (top curve). β =0.8. Full size image Figure 4: Evolutionary simulation results for a decreasing best-response case not covered by the analytic model. Benefits and cost are B ( x , y )=2( x + y )/[0.5+ x + y ] and C v ( x )=0.1(1+4 v ) x 1.5 . ( a ) Population mean values of m , δ and λ (see equation (1)), ( b ) population mean values of the average payoff over all 20 rounds (top curve) and effort on the 20th round (bottom curve). β =0.8. Full size image We have compared mean population efforts and fitness with and without reputation, where the reputation of an individual is a weighted average of their previous efforts. For reputation to have an effect, there have to be differences in the efforts of individuals. Otherwise, at any monomorphic Nash equilibrium, all individuals would expend the same effort and have the same reputation. There would then be no need to respond to the reputation of partner and thus no selection pressure to maintain a response. Furthermore, to make it worth responding to reputation, reputation has to convey information, that is, past efforts have to be partial predictive of current effort. We have achieved both of these characteristics by allowing individuals to vary in type, where the cost paid for a given level of effort increases with type. Costs are such that for a given effort of the opponent the optimal effort of an individual is a strictly decreasing function of the type of the individual. This produces the necessary variation in effort and hence reputation. Furthermore, since the type does not change between rounds, previous efforts are positively correlated with current effort, so that reputation is informative. Note that since reputation is only allowed to depend on the previous efforts of an individual, and not on the reputations of the partners of the individual, which vary, the reputation of an individual varies stochastically, and is not a perfect predictor of current effort. Previous work [7] , [8] on the negotiation of efforts in the repeated interactions between two individuals provides an additional reason to consider variation in type. By direct analogy with the analysis of negotiated efforts, there would be infinitely many neutrally stable Nash equilibria if all individuals were the same type [8] . Variation in the type removes this degeneracy and results in a unique Nash equilibrium within the class of linear response rules provided that the specific quadratic costs and benefits that are analysed in this manuscript are assumed. This Nash equilibrium is also ES against invasion by other linear response rules [7] . Our analysis restricts attention to versions of the snowdrift game; two individuals contribute effort to a common good, but at a cost to themselves. Unlike some previous work on games of this form [9] , we restrict attention to the case where the unique ESS without reputation is convergence stable. A crucial property of the games that we consider is that the effort of an individual that maximizes the payoff on a single round is a monotone function of the effort of opponent. There are then two distinct cases; that when the best effort increases with opponent’s effort and when it decreases with opponent’s effort. Our results can, perhaps, best be understood from the evolutionary simulations in Figs 2 , 3 , 4 . Consider first the case where best efforts are an increasing function of partner’s effort ( Figs 2a,b and 3 ). Since there is a positive correlation between the reputation of a partner and their current effort, the higher the reputation of the partner the greater their predicted effort in the current round. Thus, to maximize the payoff in the current round, an individual should increase their effort as the reputation of partner increases (since best efforts are increasing). Thus, when reputations are allowed, we expect λ to evolve to be positive, as occurs in the figures. Once population members evolve positive values of λ , future partners of an individual will tend to increase their effort as the current effort of the individual increases. Thus, it is worth the individual increasing effort on each round so as to benefit from this future behaviour, which leads to an increase in the evolved mean population effort. This increase in the cooperative behaviour of population members increases mean population fitness. When best efforts are a decreasing function of partner’s effort ( Figs 2c,d and 4 ), to maximize the payoff in the current round an individual should decrease their effort as the reputation of partner increases (since best efforts are decreasing). Thus, when reputations are allowed, we expect λ to evolve to be negative, as occurs in the figures. Once population members evolve negative values of λ , future partners of an individual will tend to increase their effort as the current effort of the individual decreases. Thus, it is worth the individual decreasing effort on each round so as to benefit from this future behaviour, which leads to a decrease in the evolved mean population effort and hence a decrease in mean population fitness. One might interpret this result as population members attempting to appear of lower quality than they really are, forcing their partners to compensate for their lack of effort [7] . In both of the above cases, the evolved level of effort is a compromise between maximizing the payoff in the current round and from future rounds. In the case of no reputation, at evolutionary stability, the effort of an individual is a decreasing function of the individual’s type ( ). This is because the marginal cost of increased effort increases with the type. As the figures show, allowing reputation accentuates the slope of the relationship between type and effort ( ). To understand this, we first consider the case where best efforts are increasing. In this case, λ * evolves to be positive. Thus, since reputation is negatively correlated with type, the effort of the partner of an individual is negatively correlated with the type of the individual. Since best efforts are increasing, this selects for an even greater rate at which the individual should decrease their effort as their type increases, that is, selects for a further increase in δ . In turn, since this steepens the negative relationship between the type and reputation, there is then selection for an even steeper relationship between an individual’s type and the effort of future partners and so on. This process does not, however, runaway, since λ *<1 and the best response to increased effort has slope <1 (inequality (8)). In the case where best efforts are decreasing, λ * evolves to be negative. Thus, since reputation is negatively correlated with type, the effort of the partner of an individual is positively correlated with the type of the individual. Since best efforts are decreasing, this selects for an even greater rate at which effort decreases as type increases and so on. Again the process does not runaway since in all our analytic models and computations λ *>−1 and the best response to increased effort has slope between −1 and 0. In our model, the effort contributed to the common good can be adjusted continuously. Previous work has considered various continuous versions of the prisoner’s dilemma game, and has demonstrated how the continuous nature of the contribution to a partner can lead to cooperative behaviour through direct reciprocity [10] , [11] , [12] , [13] . Here we have been concerned with a form of indirect reciprocity. However, our feedback mechanism does not enhance cooperation through indirect reciprocity in continuous versions of the prisoner’s dilemma, even if type were included. This is because the payoff for a single round of the prisoner’s dilemma is maximized by contributing zero effort regardless of the behaviour of the partner; the only reason to cooperate is to establish a reputation and hence gain benefit from others in the future. In the mechanism that we present, the fact that the level of effort put into the common good varies with the expected effort of the opponent is crucial. As in the seminal work of Nowak and Sigmund [3] on indirect reciprocity for the prisoner’s dilemma game, our analysis is based on reputations that are formed through first-order assessment: the reputation of an individual depends only on the actions of that individual and not on the reputation of the opponents of the individual. However, it does differ from that in Nowak and Sigmund in a key respect; the effort of an individual depends on the individual’s own type as well as the reputation of partner. The mechanism proposed by Nowak and Sigmund can produce persistent cooperative behaviour when individuals play the prisoner’s dilemma [14] , [15] , [16] . However, the mechanism is not evolutionary stable [17] , [18] and it has been argued that more cognitively demanding [19] higher order forms of reputation are needed [20] , [21] . Here we have demonstrated a robust and ES mechanism based only on first-order reputation that can affect levels of cooperation in games that are more relaxed [9] than the prisoner’s dilemma. Future work might extend or modify our model in various ways. In our model, an individual responds to their own type, but does not explicitly respond to their own reputation. One modification might be to consider an explicit response to own reputation. Since at evolutionary stability the mean reputation of an individual is a strictly decreasing function of their type, this suggests that this modification would not produce radically different results, but a formal analysis is needed to determine this. Another modification might allow reputation to be higher order; specifically to also depend on the reputation of the recipient of help. Again, it may be that this would not radically alter conclusions, since in our formulation reputation acts as an honest signal of quality (with noise) at evolutionary stability. Perhaps the main effect of taking this into account would be to reduce the noise, particularly when the memory factor β is small, but again a formal analysis is required. The basic game We assume a large (infinite) population. Each population member plays a series of rounds of a two-player game, where each round is against a different randomly assigned opponent. The fitness of a population member is a constant plus the average payoff obtained over many rounds. Individuals differ in their type, v , which specifies the cost paid for a given level of effort. Type is not genetically determined but is set during development, so that over the population there is a spread of types. The type V of a randomly selected population member has mean μ = E { V } and variance σ 2 = Var { V }. Type is set independently for each population member during development before the first round is played and does not change from then on. All figures presented assume that the type is uniformly distributed between 0 and 1. During each round of the game, each player must choose a non-negative level of effort. This choice is made before the effort of the partner is known (a sealed bid situation). If an individual of type v expends effort x , then their payoff in the round is when opponent expends effort y . Here the benefit B ( x , y ) is a common to both players (that is, B ( x , y )= B ( y , x ) for all x , y ) and is an increasing but decelerating function of the effort of each. The cost of effort, C v ( x ), is an increasing and accelerating function of x for each type v . The marginal cost of extra effort increases as type increases, that is, We may, therefore, think of the quality of an individual as decreasing with their type. We also assume that benefits are increasing but decelerating with effort, that is, and Finally, we assume that Consider the best effort of an individual of type v in a single round of the game when opponent expends effort y . If this focal individual expends effort x , the payoff is H v ( x )= B ( x , y )− C v ( x ). By inequality (5) and since C v ( x ) is accelerating we have so that the function H v ( x ) has a unique maximum. Let denote the value of x at which this maximum occurs. Then, assuming this maximum occurs at an internal value, we have , that is, Differentiating with respect to y and rearranging gives By assumption, C v and − B are accelerating functions so that the denominator of this expression is positive. Thus, By inequalities (5) and (6), we can also see that Special case when all individuals have the mean type Suppose that all individual have the mean type μ and there is no reputation. Assume that there is a unique Nash equilibrium effort x ** that satisfies . Then the above assumptions guarantee thatx i This effort is also an ESS. (This follows since best efforts are unique.) ii The ESS is convergence stable. (This follows from inequality (8) and standard results on continuous stability [22] .) iii There is no other Nash equilibrium effort. (This follows since inequality (8) holds for all y .) The parameter is crucial to our analysis. By definition, when J >0, the value of increasing one’s own effort increases as the partner’s effort increases. Condition (7) shows that Thus, when J >0, to maximize the payoff in a single round of the game, it is optimal to increase one’s own effort as the partner’s effort increases. Conversely, it is optimal to decrease effort when J <0. We refer to J as the interaction parameter. Reputation formation If an individual of reputation R expends effort Z , their reputation is updated to where the parameter β satisfies 0≤ β <1. When β =0, the reputation of this individual is the effort it contributed on the previous round. As β increases, previous efforts are weighted more heavily. When the number of previous rounds of interaction is large, reputation approximates the average effort over these rounds when β is close to 1. Quadratic approximation Our analytic analysis of the effect of type and reputation assumes a special form for the cost and benefits. The cost function is taken to be of the form where α is a positive parameter. Because of the term vx , the marginal cost of extra effort increases as type increases as is required by equation (3). Since α is positive, the term is an accelerating cost that is paid independently of the type. We Taylor series expand the function B ( x , y ) about ( x **, x **), ignoring terms of order 3 and above. In general, we can write this expansion as We assume that b 1 >0 so that inequality (4) is satisfied. In fact, for convenience (see Supplementary Methods ), we assume the stronger condition 0< μ < b 1 . To ensure condition (5) holds, we assume that B 2 >0. To ensure that condition (6) holds, we assume that J < B 2 . For convenience, we further restrict J so that | J |< B 2 . Given these approximations, the payoff to an individual of type v that expends effort x when partner’s effort is y is Of course, this approximation will fail for large deviations from ( x **, x **). In particular, when B ( x , y ) is given by equation (12), this function will decrease as x increases for x sufficiently large. However, there will be selection against such high levels that will typically maintain efforts in the range in which B ( x , y ) is still increasing as x increases. Evolutionary simulations Evolutionary simulations assume an asexual haploid population with discrete, non-overlapping generation. In each generation, the population size is N =2 14 =16,384. Each population member is characterized by the three genetically determined quantities m , δ and λ . An individual with these allelic values expends effort if they are type v and the current opponent has reputation r . In each generation, individuals are assigned a type value, chosen independently from a uniform distribution on the interval (0, 1); so that μ =0.5. Each individual starts with reputation r 0 =0. Population members are then paired up to play round 1. Reputations are updated and population members are paired up to play round 2 and so on. When updating reputation, the reputation after n rounds, r n , is given by where x n is the effort on this round. There are a total of 20 rounds per generation. The fitness of an individual is taken to be 1 plus the average payoff obtained over these 20 rounds. For computational efficiency, pairing is not completely at random. Instead the population is subdivided into 64 demes each containing 256 individuals at the start of a generation, and all partners of an individual are chosen independently and at random from the other members of the individual’s deme. The next generation is formed by choosing each new individual to be the offspring of a member of the previous generation, where this parent is chosen with a probability proportional to their fitness. Each of the N members of this new generation are chosen independently. Each offspring inherits the mutated alleles of its parent. Mutation acts so that if the parent allele value is q then the mutated value is q +0.1(Δ q −0.5) 3 , where Δ q ~ U (0,1). Mutations on different alleles are independent. How to cite this article : McNamara, J. M. and Doodson, P. Reputation can enhance or suppress cooperation through positive feedback. Nat. Commun. 6:6134 doi: 10.1038/ncomms7134 (2015).